Trans-ethnic genome-wide association study of colorectal cancer identifies a new susceptibility locus inVTI1A The genetic basis of sporadic colorectal cancer (CRC) is not well explained by known risk polymorphisms. Here we perform a meta-analysis of two genome-wide association studies in 2,627 cases and 3,797 controls of Japanese ancestry and 1,894 cases and 4,703 controls of African ancestry, to identify genetic variants that contribute to CRC susceptibility. We replicate genome-wide statistically significant associations ( P <5 × 10 −8 ) in 16,823 cases and 18,211 controls of European ancestry. This study reveals a new pan-ethnic CRC risk locus at 10q25 (rs12241008, intronic to VTI1A ; P =1.4 × 10 −9 ), providing additional insight into the aetiology of CRC and highlighting the value of association mapping in diverse populations. Colorectal cancer (CRC) is the third most common cancer and the second leading cause of cancer deaths in the United States. Genetics is known to play an important role in CRC susceptibility [1] . However, genome-wide association studies (GWASs), mostly conducted in European-descent populations, have only identified 30 common risk variants (22 independent loci) for CRC, markedly fewer than for prostate or breast cancer. To discover additional risk loci for this cancer, we combine, via a meta-analysis, two GWASs of CRC in populations of Japanese and African American ancestry. The top associations for single-nucleotide polymorphisms (SNPs) in VTI1A are replicated in European-descent populations. 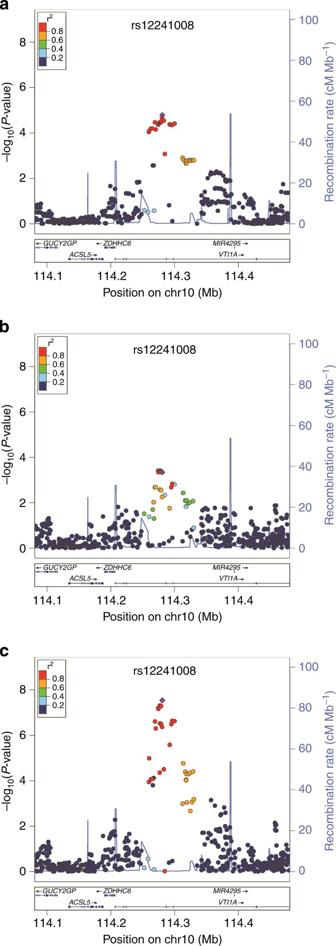Figure 1: RegionalP-value plots for the new colorectal cancer susceptibility locus at 10q25. Results in the Japanese (a) (n=6,424), African Americans (b) (n=6,595) and in the combined data (Japanese and African Americans) (c) are displayed. The SNP with the smallestP-value from meta-analysis in the combined data (n=13,019), rs12241008, is shown as a purple diamond.r2is in relation to this SNP from the 1000 Genomes Project in East Asians (a,c) or in Africans (b). The plots were generated using LocusZoom26. In the first GWAS, Japanese samples ( n =6,424) were identified from the Multiethnic Cohort study (MEC), the Colorectal Cancer Family Registry (CCFR), the Japan Public Health Center cohort study (JPHC) and three case–control studies in Hawaii (CR2&3) and in Fukuoka and Nagano, Japan ( Supplementary Table 1 ). Blood leukocyte DNA samples were genotyped on the Illumina 1M-Duo or the Illumina 660W-Quad arrays, yielding, after quality control (QC) procedures, data for 323,852 SNPs available for all Japanese samples (see Methods and Supplementary Methods ). Un-typed markers or markers with partly missing values were imputed with BEAGLE [2] using East Asians from the 1000 Genomes Project (phase 1, release 3) as the reference panel. The second GWAS of African American samples ( n =6,597) ( Supplementary Table 2 ) were identified from the MEC, CCFR, the Southern Community Cohort Study (SCCS), the MD Anderson Cancer Center, the University of North Carolina CanCORS study (UNC-CanCORS) and Rectal Cancer Study (UNC-Rectal), and from the Prostate, Lung, Colorectal and Ovarian Cancer Screening (PLCO) Trial. African American samples were genotyped using the Illumina 1M-Duo bead arrays (except 170 PLCO subjects on Illumina Omni 2.5M). Imputation was performed with BEAGLE using Europeans and Africans from the 1000 Genomes Project (phase 1, release 3) as reference panels. Over 4.2 million genotyped or imputed autosomal markers were available for both studies. In both GWASs, cases and controls were well matched with regard to genetic ancestry based on principal component (PC) analyses (Methods and Supplementary Figs 1 and 2 ). We used logistic regression within each ethnic group to test for the association of SNP dosage with CRC risk, adjusting for age at blood draw, sex and the first four PCs. The genomic control [3] inflation factor ( λ ) was 1.04 for each individual study, indicating little effect of population stratification after controlling for global ancestries ( Supplementary Fig. 3 ). After combining the two GWASs, we observed three SNPs in the VTI1A gene on chromosome 10q25 to be statistically significant at the genome-wide significance level ( P <5 × 10 −8 ; Fig. 1 ; Table 1 ). The strongest association was for rs12241008 (114,280,702 bp) (odds ratio (OR)=1.19, 95% confidence interval (CI) 1.12–1.26, P =2.9 × 10 −8 , allele frequency 0.19 and 0.25 in African Americans and Japanese, respectively), with highly consistent associations in both populations ( I 2 =0). The other two SNPs, rs7894915 (114,277,039 bp, P =4.8 × 10 −8 ) and rs10082356 (114,278,181 bp, P =4.9 × 10 −8 ), were in high linkage disequilibrium (LD) with rs12241008 ( r 2 from 0.80 to 1.0 in East Asians, Africans and Europeans), with risk estimates almost identical to those for rs12241008 ( Supplementary Tables 3 and 4 ). This locus has not previously been reported to be associated with CRC. Figure 1: Regional P -value plots for the new colorectal cancer susceptibility locus at 10q25. Results in the Japanese ( a ) ( n =6,424), African Americans ( b ) ( n =6,595) and in the combined data (Japanese and African Americans) ( c ) are displayed. The SNP with the smallest P -value from meta-analysis in the combined data ( n =13,019), rs12241008, is shown as a purple diamond. r 2 is in relation to this SNP from the 1000 Genomes Project in East Asians ( a , c ) or in Africans ( b ). The plots were generated using LocusZoom [26] . Full size image Table 1 Most strongly associated SNP in the new colorectal cancer susceptibility locus 10q25. Full size table We subsequently replicated these associations in two large CRC consortia of European-descent populations (allele frequency 0.09): Colorectal Transdisciplinary Study (CORECT) with 7,561 cases and 6,328 controls from eight participating studies (combined OR=1.09, P =0.036, Table 1 ), and the Genetics and Epidemiology of Colorectal Cancer Consortium (GECCO) with 9,262 cases and 11,883 controls from 18 participating studies (combined OR=1.09, P =0.018, Table 1 ). The combined P -value for rs12241008 in the Japanese, African Americans and Europeans was 1.4 × 10 −9 (OR=1.13, 95% CI 1.09–1.18). A meta-analysis using individual study-level statistics yielded similar results ( P =1.5 × 10 −9 ). Although risk estimates were consistent across individual studies ( I 2 =8%, P het =0.35, d.f.=27) (see the forest plot in Supplementary Fig. 4 ), there was some evidence for heterogeneity in effects across ethnic groups ( I 2 =53%, P het =0.12, d.f.=2). This possible heterogeneity in effects, along with the low allele frequencies observed in European-descent populations (and therefore low power), could partially explain why previous GWASs in Europeans failed to identify this locus, and thus emphasizes the importance of conducting GWASs in ethnically diverse populations. Similar results were observed for rs7894915 and rs10082356 when the data were combined with the European-descent GWASs ( P =1.6 × 10 −9 and 1.5 × 10 −9 , respectively). Nine other SNPs in this region (located within 12 kb in the same LD block as rs12241008 in East Asians, Africans and Europeans, Supplementary Fig. 5 ) also had P -values<5 × 10 −8 when all data were combined ( Supplementary Tables 3 and 4 ). However, the strongest association signal was still with rs12241008 ( Supplementary Fig. 5 ) and none of the other nearby SNPs within 200 kb represented an independent signal after conditioning on rs12241008 in the African American and Japanese GWASs. Results for these 12 SNPs were similar (change in OR <1.2%) with or without adjustment for local ancestry estimates among African Americans (Methods). There was no important heterogeneity in ORs in the Japanese or the African American data by anatomical site (colon versus rectal cancer) ( P -values>0.74), by stage (regional/distant versus local/ in situ ) ( P -values>0.6), by age of diagnosis ( P -values>0.7) or by sex ( P =0.04 in African Americans and 0.80 in Japanese) for the most significant marker rs12241008 (stratified analysis results are in Supplementary Table 5 ). No association reached the genome-wide significance threshold (5 × 10 −8 ) in the Japanese GWAS when analysed separately. One SNP on chromosome 7, rs79453636, passed this threshold ( P =2.9 × 10 −8 ) in the African American study ( Supplementary Fig. 3 ). However, this association was not replicated ( Supplementary Table 6 ) in the Japanese or in the combined European-descent data ( P -values>0.15). Out of 30 known CRC susceptibility SNPs, 27 were available for analysis in the Japanese study and 23 (85%) effects were in the same direction as in the original GWAS reports ( Supplementary Table 7 ). Replication and fine-mapping of the known risk loci in the African American study was summarized previously [4] . Twelve out of the 27 associations were replicated in the meta-analysis of the Japanese and African American data ( P <0.05) and 23 risk estimates were directionally consistent with those originally reported ( Supplementary Table 7 ). Considerable heterogeneity in disease risk between the two ethnic groups ( I 2 >50%) was observed for six SNPs ( Supplementary Table 7 ). The three genetic variants with the strongest association with CRC, rs12241008, rs7894915 and rs10082356, are located in intron 3 of the VTI1A gene, which encodes vesicle transport through interaction with t-SNAREs 1A. VTI1A is involved in regulating insulin-stimulated trafficking of secretory vesicles enriched with both GLUT4 (glucose transporter) and Acrp30 in adipocytes [5] ; it also plays key roles in neuronal development [6] and in selectively maintaining spontaneous neurotransmitter release [7] . A recent GWAS in never-smoking Asian women has identified rs7086803 in intron 7 of VTI1A as a lung cancer susceptibility variant (218 kb from and not in LD with rs12241008) [8] . Interestingly, a gene fusion product, VTI1A-TCF7L2 , was identified in colorectal tumours and shown to promote anchorage-independent growth of cultured tumour cells [9] . The fusion occurs between VTI1A exon 3 (chr10: 114,220,869) and TCF7L2 exon 4 (chr10: 114,760,545) and results in the deletion of both the intron 3 CRC and intron 7 lung cancer risk variants. No coding variant is in LD with the top three SNPs. Among the three VTI1A SNPs associated with CRC in this study, rs7894915 and rs10082356 lie in predicted transcriptional regulatory regions, suggesting enhancer and promoter regulatory activities across multiple cell lines ( Supplementary Table 8 ) [10] . We explored regulatory effects of the SNPs correlated with rs12241008 in a cis -expression quantitative trait loci analysis in 40 paired colon adjacent-normal and tumour tissue samples from European descent patients [11] . Among the SNPs in high LD ( r 2 >0.8) with rs12241008 in East Asians, the intronic SNP rs7081965 (alleles: A/T) affected VTI1A expression ( P =0.003) in colon tumour tissue. Rs7081965 is also in considerable LD with rs12241008 in Africans ( r 2 =0.21, | D ′|=0.88) and in Europeans ( r 2 =0.24, | D ′|=1) in the 1000 Genomes data. Although the association of rs7081965 with CRC was not statistically significant in this study (OR=1.09 for allele T , P =8.2 × 10 −6 from the three ethnic groups combined), these results provide an interesting lead for future functional investigations. In summary, this trans-ethnic GWAS identified a new CRC susceptibility locus at 10q25 with directionally consistent associations across three ethnic/racial populations, providing additional insight into the genetic architecture of CRC. Further work is needed to dissect this genetic signal and to conduct functional studies to uncover the mechanisms underlying this association. Japanese subjects and QC on genotypes Details on study design and basic characteristics for each study are provided in Supplementary Methods . Briefly, 1,703 MEC Japanese American subjects were genotyped by the Broad Genotyping Center on the Illumina 1M-Duo Array and 1,602 (803 cases, 799 controls) passed their initial QC filters. To maximize sample size, initially ‘failed’ samples on five plates were re-clustered with a customized genotype calling algorithm—this step recovered 42 additional MEC subjects (23 cases, 19 controls), although not all SNPs on the array were preserved. To increase statistical power and to provide a larger control pool, 1,033 prostate cancer-free men and 808 breast cancer-free women genotyped on the Illumina 660W‐Quad platform were drawn from the MEC prostate cancer [12] and breast cancer [13] studies, respectively. Japanese from the following studies were all genotyped on the Illumina 1M-Duo array by the University of Southern California (USC) Epigenome Center: 697 from CCFR (384 cases, 313 controls), 155 cases from CR2&3, 1,463 from Fukuoka, Japan (685 cases, 778 controls), 212 from Nagano, Japan (106 cases, 106 controls) and 1,332 from JPHC (670 cases, 662 controls). In general, all genotyped samples were examined and excluded according to the following: (1) call rates<90%, 95% or 97% depending on the batches, (2) missing on basic covariates (age, sex or disease status), (3) gender mismatch, that is, the reported sex was different from that estimated based on X chromosome inbreeding coefficient F , calculated by PLINK ( http://pngu.mgh.harvard.edu/~purcell/plink/ ), (4) ethnicity outliers, that is, subjects fell out of the Japanese cluster (by visual inspection) on PC plots, where PCs were derived for study subjects as well as unrelated HapMap CEU, YRI and JPT samples with our own R program (The Comprehensive R Archive Network http://www.r-project.org/ ), based on about 20k SNPs with inter-marker distance>100 kb, and (5) close ( ⩾ 2nd degree) relatives, where relationships were derived from estimated probabilities of sharing 0, 1 or 2 alleles based on genomic data (calculated by PLINK), and relatives were removed in the following order: subjects with most relatives, controls and subjects with lower call rates. All cases were verified by histological records to have invasive carcinoma of the colon or rectum. More details on genotype QC can be found in Supplementary Methods . After QC, the following subjects were retained in analysis: 3,094 from the MEC (797 cases, 2,297 controls), 285 from CCFR (276 cases and 9 controls), 134 cases from CR2&3, 1,411 from Fukuoka, Japan (662 cases, 749 controls), 207 from Nagano, Japan (105 cases, 102 controls) and 1,293 from the JPHC (653 cases, 640 controls). African American subjects and QC on genotypes Sample collection and genotyping QC have been described in detail elsewhere [4] and in Supplementary Methods . We genotyped 7,168 African American samples from six studies/centres: the MEC (442 cases, 4,620 controls), CCFR (999 cases, 290 controls), SCCS (164 cases, 160 controls), the MD Anderson Cancer Center (189 cases), UNC-CanCORS (84 AA cases) and UNC-Rectal (112 cases, 108 controls) on the Illumina 1M-duo platform. QC procedures for all subjects were similar to the criteria described for the Japanese study subjects. Included in analysis were 6,427 subjects (4,609 controls, 1,818 cases) on 1,049,327 markers. We also included 170 PLCO samples (76 cases, 94 controls) that were previously genotyped on the Illumina Omni 2.5M array and pre-filtered by the NCI genotyping centre for analysis (527,383 markers that overlapped with other studies). Overall, 6,597 subjects (1,894 cases, 4,703 controls) were used in association testing. Supplementary Table 2 shows the distribution of subjects by participating study. Imputation Prediction of un-typed or partly genotyped SNPs was performed with BEAGLE 3.3 (ref. 2 ) using the 1000 Genomes Project (phase 1, release 3) East Asians as reference panels for the Japanese data and Europeans and Africans for the African American data. Imputation was performed separately for the two ethnic groups with all cases and controls combined. Markers with minor allele frequencies<0.005 in reference panels were excluded from imputation. For the African American data, 10,050,748 markers with imputation accuracy R 2 >0.8 were kept for association analysis; for Japanese data, 4,266,108 markers with imputation R 2 >0.95 were retained. Altogether, 4,276,079 autosomal genotyped or imputed markers were available in both populations for meta-analysis. Analysis of the Japanese and African American GWASs PCs were calculated as in EIGENSTRAT [14] with our own R program, including unrelated HapMap CEU, YRI and JPT samples as population controls. Ethnicity outliers were identified on PC plots by visual inspection and subsequently removed. Pair-wise PC plots suggested that the first two PCs were most informative for global ancestry and the distribution of PCs was similar among all cases and controls in both Japanese and African Americans ( Supplementary Figs 1 and 2 ). Logistic regression of CRC on allelic dosage with adjustment for age at blood draw, sex and the first four PCs was performed to obtain OR estimates and 95% CI of per increase in allele count with PLINK, where age was grouped as <55 years, 5-year intervals from 55 to 80 and ⩾ 80 years. The genomic control factor ( λ ) was estimated from the median of the χ 2 statistics divided by 0.456. Heterogeneity of genetic effects by site (colon versus rectal cancer, mutually exclusive), stage (regional/distant versus local/ in situ ) and age at diagnosis (≤55 versus >55 years) was tested in a case-only analysis. Effect modification by sex was assessed comparing the model with and without the cross-product term. These and additional stratified analyses by site, stage, age at diagnosis and sex were adjusted for age at blood draw, sex (where appropriate), the first four PCs and BMI. Conditional analyses were performed to examine the independence of association signals in the chromosome 10 region, conditioning on the SNP with the smallest P -value. Significance of the additional contribution by other SNPs was calculated based on a likelihood ratio test. These analyses were carried out using SAS 9.3. Local ancestry estimation for African Americans The percentage of African ancestry (0, 50 or 100%, that is, half of the estimated number of African chromosomes) was inferred for each participant at the putative CRC risk locus on chromosome 10 (±250 kb) with the LAMP program v2.4 (ref. 15 ). To summarize local ancestry, for each individual we averaged across all local ancestry estimates that are within the region. The effect of local ancestry was evaluated by examining the relative change in ORs with and without adjustment for local ancestry in logistic regression. CORECT study for replication The CORECT study meta-analysis was conducted using germline DNA in the Molecular Epidemiology of Colorectal Cancer study (MECC) (set 1: 484 cases and 498 controls; set 2: 1,120 cases and 820 controls), CCFR (set 1: 1,977 cases and 999 controls; set 2: 1,660 cases and 1,393 controls), Kentucky case–control study (1,038 cases and 1,134 controls), Newfoundland case–control study (548 cases and 538 controls), American Cancer Society CPS II nested case–control study (ACS/CPSII, 539 cases and 469 controls) and the Melbourne nested case–control study (195 cases and 477 controls). All subjects were self-reported whites. The majority of the studies were genotyped using the Affymetrix Axiom CORECT Set containing ~1.3 million SNPs and indels on two physical genotyping chips ( Supplementary Table 3 ). Genotype data were screened based on filters such as call rates, concordance rates, sample relatedness and ethnic outliers. IMPUTE2 (ref. 16 ) was used to impute missing genotypes based on the cosmopolitan panel of reference haplotypes from Phase I of the 1000 Genomes Project. Imputed genotypes were screened based on stringent imputation quality and accuracy filters (info ⩾ 0.7, certainty ⩾ 0.9, concordance ⩾ 0.9 between directly measured and imputed genotypes after masking input genotypes for genotyped markers only). Associations between genetic variants and CRC risk were tested using a log-additive genetic model within each study, allowing for study-specific adjustment for age, sex, study centre, genotyping batch and 2–4 PCs. More details of each participating study can be found in Supplementary Methods . GECCO study for replication The GECCO GWAS consortium has been described before [17] , [18] , [19] . The consortium consisted of European-descent participants within the French Association Study Evaluating RISK for sporadic CRC (ASTERISK, 948 cases and 947 controls); CR2&3 (87 cases and 125 controls); Darmkrebs: Chancen der Verhütung durch Screening (DACHS set 1: 1,710 cases and 1,707 controls; DACHS set 2: 675 cases and 498 controls); Diet, Activity, and Lifestyle Study (DALS set 1: 706 cases and 710 controls; DALS set 2: 410 cases and 464 controls); Health Professionals Follow-up Study (HPFS set 1: 227 cases and 230 controls; HPFS set 2: 176 cases and 172 controls); MEC (328 cases and 346 controls); Nurses’ Health Study (NHS set 1: 394 cases and 774 controls; NHS set 2: 159 cases and 181 controls); Ontario Familial Colorectal Cancer Registry (OFCCR, 650 cases and 522 controls); Physician’s Health Study (PHS, 382 cases and 389 controls); Postmenopausal Hormone study (PMH, 280 cases and 122 controls); Prostate, Lung, Colorectal, and Ovarian Cancer Screening Trial (PLCO set 1: 533 cases and 1,976 controls; PLCO set 2: 486 cases and 415 controls); VITamins And Lifestyle (VITAL, 285 cases and 288 controls); and the Women’s Health Initiative (WHI set 1: 470 cases and 1,529 controls; WHI set 2: 1,006 cases and 1,010 controls). All individual studies were genotyped on Illumina arrays on 240k–730k markers and went through rigorous QC. The genotype data were imputed to increase the density of genetic variants. The haplotypes from the 1000 Genomes Project Phase I were used as the reference panel. Logistic regression of CRC on SNP dosage effect on CRC risk was performed with adjustment for age, sex (when appropriate), centre (when appropriate), smoking status (PHS only), batch effects (ASTERISK only) and the first three PCs from EIGENSTRAT [13] to account for population substructure within each individual study. Additional details on sample collection, genotyping, QC and statistical methods are provided in Supplementary Methods . All samples were collected with informed consent and all procedures were approved by the Human Research Institutional Review Boards (IRBs) at relevant institutions. Specifically, the study protocols of the Japanese and African Americans’ GWASs were approved by the University of Hawaii Human Studies Program and University of Southern California IRB, the IRB in the National Cancer Center, Japan, the Ethics Committee of Kyushu University Faculty of Medical Sciences, the University of North Carolina IRB, Vanderbilt University IRB, the Fred Hutchinson Cancer Research Center IRB and the MD Anderson Cancer Center IRB. The GECCO portion of this work was approved by the Fred Hutchinson Cancer Research Center IRB. The University of Southern California Health Sciences IRB approved all elements of the CORECT study. Meta-analysis A fixed-effect model with inverse variance weighting implemented in METAL [20] was used to combine the results from the Japanese and the African American studies and for further combining with replication studies. Heterogeneity measure I 2 was calculated and Cochran’s Q statistic to test for heterogeneity was calculated [21] . For the 12 top hits in the VTI1A region at 10q25 (see text), OFCCR in GECCO was excluded because these SNPs did not pass the quality filters in this substudy ( Table 1 , Supplementary Table 4 and Supplementary Fig. 4 ). In Supplementary Fig. 5 , SNPs that passed the filters in OFCCR were included whenever applicable. How to cite this article: Wang, H. et al . Trans-ethnic genome-wide association study of colorectal cancer identifies a new susceptibility locus in VTI1A . Nat. Commun. 5:4613 doi: 10.1038/ncomms5613 (2014).